Chromatin decompaction by the nucleosomal binding protein HMGN5 impairs nuclear sturdiness In most metazoan nuclei, heterochromatin is located at the nuclear periphery in contact with the nuclear lamina, which provides mechanical stability to the nucleus. We show that in cultured cells, chromatin decompaction by the nucleosome binding protein HMGN5 decreases the sturdiness, elasticity and rigidity of the nucleus. Mice overexpressing HMGN5, either globally or only in the heart, are normal at birth but develop hypertrophic heart with large cardiomyoctyes, deformed nuclei and disrupted lamina and die of cardiac malfunction. Chromatin decompaction is seen in cardiomyocytes of newborn mice but misshaped nuclei with disrupted lamina are seen only in adult cardiomyocytes, suggesting that loss of heterochromatin diminishes the ability of the nucleus to withstand the mechanical forces of the contracting heart. Thus, heterochromatin enhances the ability of the nuclear lamina to maintain the sturdiness and shape of the eukaryotic nucleus; a structural role for chromatin that is distinct from its genetic functions. Dynamic changes in the organization and spatial localization of chromatin play a central role in regulating the fidelity of gene expression, in the maintenance of genomic stability and in the progression of cellular processes such as the cell cycle and differentiation [1] , [2] , [3] , [4] . For example, gene silencing is often associated with chromatin condensation into lamina-associated domains at the nuclear periphery, while gene reactivation is associated with chromatin decompaction and relocation towards the centre of the nucleus [4] , [5] . The nuclear lamina underlining the inner nuclear membrane is in contact with heterochromatin and affects chromatin organization and function [6] , [7] , [8] , [9] . Although transcriptional silent heterochromatin tends to be sequestered at the nuclear periphery, association with nuclear lamina is not an absolute requirement for heterochromatin maintenance since in rod photoreceoptor cells of nocturnal animals, and in mutant mice lacking components of the nuclear lamina, heterochromatin localizes towards the nuclear centre [10] , [11] . Likewise, in yeast cells which lack a distinct lamina, components of the nuclear envelope affect nuclear shape and chromatin organization [12] , [13] . Thus, the function of condensed heterochromatin at the nuclear periphery is not fully understood. To gain insights into the function of heterochromatin, we reduced chromatin compaction by overexpressing the nucleosome binding protein HMGN5, in cells and mice. HMGN5 is a member of the high mobility group N (HMGN) protein family, which binds dynamically to nucleosomes without any specificity for the underlying DNA sequence and reduces the interaction of H1 with chromatin [14] . Histone H1, the most abundant family of nucleosome binding proteins, plays a major role in the formation and stabilization of compact chromatin structures [15] , while HMG proteins have an opposing effect and destabilize higher order chromatin compaction [16] , [17] . The HMGN5 variant efficiently counteracts the chromatin-condensing activity of histone H1 and as a consequence, its overexpression leads to global chromatin decompaction [14] including loss of peripheral chromatin. Thus, we decompacted chromatin by reducing the chromatin residence time of H1. Our analysis of cells in tissue culture and transgenic mice indicate that loss of heterochromatin weakens the structure of the nucleus and leads to phenotypes that resemble cells and mice with defective lamina components. We suggest that the heterochromatin serves to maintain the structural integrity of the nucleus by enhancing the ability of the nuclear lamina to maintain the sturdiness and shape of the nucleus; a structural role for chromatin that is not related to gene expression. Chromatin decompaction diminished nuclear sturdiness Previous analyses indicated that upregulation of HMGN5 leads to global chromatin decompaction [14] . During these studies, we noted that upregulation of HMGN5 leads not only to chromatin decompaction, but also to nuclear blebbing, in all the cell lines we have tested ( Fig. 1a , Supplementary Fig. 1a ). HMGN5-mediated chromatin decompaction is due to reduced H1 binding to nucleosomes [14] and is not associated with changes in the levels of H1 ( Supplementary Fig.1b ) or of histone modifications that mark heterochromatin or inactive promoters such H3K9me3, H3K9me2 and H3K27me3 ( Fig. 1b ). In mouse embryonic fibroblasts (MEFs) and thyroid epithelial cell line CAT413, 17% of the HMGN5–green fluorescent protein (GFP) transfected cells exhibited noticeable blebbing; over 50% of the blebs were classified as either moderate (++) or severe (+++). In contrast, <7% of the cells expressing GFP or similar amounts ( Supplementary Fig.1c ) of the HMGN5S17,21E mutant (HMGN5-SE), that does not bind to nucleosomes and does not decompact chromatin efficiently [14] contained blebs; over 70% of these were classified as small, and none as severe ( Fig. 1d ). The HMGN5-induced nuclear blebs contain lamin A/C but lack lamin B1 ( Fig.1a ) and thus resemble blebs seen in cells with mutated lamins and defective lamina organization [8] , [18] ; yet, the expression of lamin A/C or lamin B1 is not affected in these cells ( Fig. 1c ). As a further test, we examined the effect of chromatin decompaction on the nuclei of MEFs with a weakened lamina, obtained from Lmna −/− mice. The analysis of MEFs obtained from Lmna −/− or their Lmna +/+ littermates [19] show that chromatin decompaction in cells with an already weakened lamina leads to synergistic effects; 40% of the HMGN5-transfected Lmna −/− cells show blebs ( Fig. 1f ). 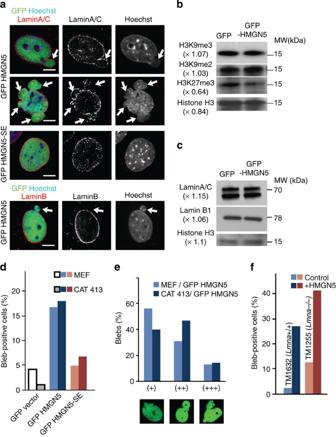Figure 1: Chromatin decompaction induced by HMGN5 overexpression leads to nuclear blebbing. (a) Cells overexpressing GFP–HMGN5, but not cells overexpressing GFP–HMGN5S17,21E (HMGN5-SE), show loss of heterochromatin (right panels) and nuclear blebs (arrows) that stain with lamin A/C, but not lamin B1. Quantitative microscopy verified that similar amounts of WT or mutant HMGN5–GFP were expressed (Supplementary Fig. 1c). Scale bar, 10 μm. (b) HMGN5-mediated chromatin decompaction does not alter the levels of histone modifications indicative of compact chromatin. Numbers in parenthesis show GFP/GFP–HMGN5 signal intensity. (c) Western blot showing that HMGN5-mediated chromatin decompaction does not alter the levels of lamin A/C or lamin B1. Numbers in parenthesis show GFP/GFP–HMGN5 signal intensity. (d) Frequency of blebbed nuclei in MEFs and CAT413 cells. For each cell type, 750 to 2,000 cells were examined. (e) Severity of blebs: (+) small extruded nuclear membrane, (++) large bleb, (+++) more than two blebs. Data shown are derived from 261 (MEF) and 239 (CAT413) GFP–HMGN5-positive cells. (f) Synergistic effects of HMGN5 overexpression and loss of lamin A on nuclear blebbing. Shown is the frequency of blebs in MEFs isolated from littermateLmna+/+andLmna−/−mice that either do or do not overexpress HMGN5. Data derived from analysis of a total of over 2,000 cells. Figure 1: Chromatin decompaction induced by HMGN5 overexpression leads to nuclear blebbing. ( a ) Cells overexpressing GFP–HMGN5, but not cells overexpressing GFP–HMGN5S17,21E (HMGN5-SE), show loss of heterochromatin (right panels) and nuclear blebs (arrows) that stain with lamin A/C, but not lamin B1. Quantitative microscopy verified that similar amounts of WT or mutant HMGN5–GFP were expressed ( Supplementary Fig. 1c ). Scale bar, 10 μm. ( b ) HMGN5-mediated chromatin decompaction does not alter the levels of histone modifications indicative of compact chromatin. Numbers in parenthesis show GFP/GFP–HMGN5 signal intensity. ( c ) Western blot showing that HMGN5-mediated chromatin decompaction does not alter the levels of lamin A/C or lamin B1. Numbers in parenthesis show GFP/GFP–HMGN5 signal intensity. ( d ) Frequency of blebbed nuclei in MEFs and CAT413 cells. For each cell type, 750 to 2,000 cells were examined. ( e ) Severity of blebs: (+) small extruded nuclear membrane, (++) large bleb, (+++) more than two blebs. Data shown are derived from 261 (MEF) and 239 (CAT413) GFP–HMGN5-positive cells. ( f ) Synergistic effects of HMGN5 overexpression and loss of lamin A on nuclear blebbing. Shown is the frequency of blebs in MEFs isolated from littermate Lmna +/+ and Lmna −/− mice that either do or do not overexpress HMGN5. Data derived from analysis of a total of over 2,000 cells. Full size image The HMGN5-mediated chromatin decompaction also leads to loss of nuclear elasticity, since in reversible swelling experiments [20] the HMGN5-overexpressing nuclei that were swollen by exposure to hypotonic solvent did not shrink when re-exposed to high salt solution, while nuclei expressing the HMGN5-SE mutant did shrink to their pre-swollen volume ( Fig. 2a ). Furthermore, chromatin decondensation in Lmna −/− nuclei leads to a total loss of elasticity; these nuclei were already fully enlarged under ‘condensed’ conditions and they neither swelled in hypotonic solutions nor shrunk when re-exposed to isotonic media ( Fig. 2d ). 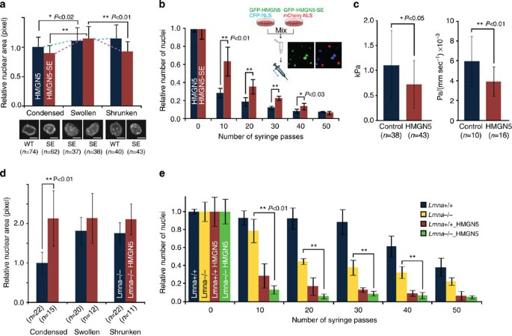Figure 2: Chromatin decompaction reduces nuclear rigidity. (a) Chromatin decompaction reduces nuclear elasticity. Shown is quantitative analysis of swelling and shrinking of nuclei transfected with either wild-type (WT) or mutant (SE) HMGN5. Scale bar, 5 μm. (b) Chromatin decompaction reduces nuclear sturdiness. Cells co-expressing either HMGN5–GFP and CFP–NLS (green and blue cells) or HMGN5S17,21E–GFP and mCherry–NLS (green and red cells) were mixed, subjected to shear by repeated passage through a G26 needle, and the remaining number of blue and red nuclei quantified. All blue and red cells were also green (seeSupplementary Fig. 2). Data shown are mean±s.d. from five independent experiments. (c) Atomic force microscopy measurements indicate that HMGN5-mediated chromatin decompaction reduces nuclear sturdiness and elasticity. (d) Synergistic effects of HMGN5 overexpression and loss of lamin A on nuclear elasticity. Shown is quantitative analysis of the effect of HMGN5 overexpression on swelling and shrinking ofLmna+/+andLmna−/−MEFs nuclei. (e) Synergistic effects of HMGN5 overexpression and loss of lamin A on nuclear sturdiness. Experiments performed as described in legend tob. s.d. from three independent experiments.Pvalues are determined by Student’st-test. **<0.01. Figure 2: Chromatin decompaction reduces nuclear rigidity. ( a ) Chromatin decompaction reduces nuclear elasticity. Shown is quantitative analysis of swelling and shrinking of nuclei transfected with either wild-type (WT) or mutant (SE) HMGN5. Scale bar, 5 μm. ( b ) Chromatin decompaction reduces nuclear sturdiness. Cells co-expressing either HMGN5–GFP and CFP–NLS (green and blue cells) or HMGN5S17,21E–GFP and mCherry–NLS (green and red cells) were mixed, subjected to shear by repeated passage through a G26 needle, and the remaining number of blue and red nuclei quantified. All blue and red cells were also green (see Supplementary Fig. 2 ). Data shown are mean±s.d. from five independent experiments. ( c ) Atomic force microscopy measurements indicate that HMGN5-mediated chromatin decompaction reduces nuclear sturdiness and elasticity. ( d ) Synergistic effects of HMGN5 overexpression and loss of lamin A on nuclear elasticity. Shown is quantitative analysis of the effect of HMGN5 overexpression on swelling and shrinking of Lmna +/+ and Lmna −/− MEFs nuclei. ( e ) Synergistic effects of HMGN5 overexpression and loss of lamin A on nuclear sturdiness. Experiments performed as described in legend to b . s.d. from three independent experiments. P values are determined by Student’s t -test. **<0.01. Full size image We also examined the fragility of the nuclei, by co-transfecting MEFs either with vectors expressing HMGN5–GFP and nuclear localization signal–cyan fluorescent protein (NLS–CFP), or with vectors expressing HMGN5-SE and NLS–mCherry ( Fig. 2b ). The cultured cells were collected, combined and repeatedly passed through a 26G needle, thereby exposing them to mechanical shear. The relative amount of blue (CFP positive) and red (mCherry positive) nuclei in the mixture provides a measure of the sturdiness of the nuclei of these cells. We verified that these nuclei were also green, an indication that they also expressed either GFP–HMGN5 or GFP–HMGN5-SE ( Supplementary Fig. 2 ). We also verified that the two cell types were of equal sturdiness since after two syringe passes all the cells were broken and released intact nuclei, an indication that the fragility of the cell is not affected ( Supplementary Fig. 1d ). After 10 syringe passes, 70% of the HMGN5-expressing nuclei, but only 40% of the HMGN5S17,21E expressing nuclei were lost ( Fig. 2b ), an indication that HMGN5 expression decreases the sturdiness of the nucleus to a greater degree than expression of the HMGN5S17,21E mutant, which does not decompact chromatin. Similar experiments with Lmna −/− and Lmna +/+ revealed that 80% of the Lmna −/− nuclei with condensed chromatin, but only 10% of the Lmna −/− nuclei with decondensed chromatin survived the shearing resulting from 10 passes through the needle. Thus, defective lamina and chromatin decompaction synergistically increase nuclear fragility ( Fig. 2e ). Likewise, atomic force microscopy (AFM) measurements at either constant or variable indentation rates [21] , [22] , revealed that chromatin decompaction led to a 31% decrease in the Young’s modulus and a 34% decrease in the viscosity of the cells ( Fig. 2c ), an indication that the nuclei of HMGN5-expressing cells were less robust than those of control cells. Together, the results suggest that the HMGN5-mediated chromatin decompaction alters the mechanical properties of the nuclear membrane in a manner similar to that seen in cells with defective lamina components, and that chromatin compaction reinforces the ability of the lamina to maintain nuclear integrity especially under mechanical stress. HMGN5 overexpression leads to impaired cardiac function Lamin A/C-deficient mice ( Lmna −/− mice) appear normal at birth [19] , [23] but develop abnormalities, including dilated cardiomyopathy [23] . In the adult mice, the cardiomyocytes nuclei are enlarged, misshapen and lack heterochromatin [23] . We find a similar phenotype in conditional transgenic mice overexpressing HMGN5–FLAG either globally, starting at E 6.5 ( Hmgn5 -TG), or only in the heart, starting at E11.5 ( Hmgn5 -hTG) ( Supplementary Fig. 3 ). Newborn Hmgn5 -TG mice express HMGN5 robustly in many tissues ( Fig. 3a , Supplementary Fig. 3d ) yet, pathological examination did not reveal any gross abnormalities in the newborn. However, the mice began dying within 1 day of birth, failed to thrive, and 85% of the mice died by the age of 6 weeks. Examination of 3-week-old survivors revealed abnormalities only in heart morphology. Similar to the lamina A/C-deficient mice [23] , Hmgn5 -TG mice had thinner ventricular walls ( Fig. 3b , Supplementary Fig. 4a ) and contained cardiomyocytes with large, misshapen nuclei with decondensed chromatin ( Fig. 3c,d ). Reverse transcription–PCR (RT–PCR) reveals a 12-fold increase of the β-myosin heavy chain (β-MHC)/α-MHC levels in the heart of 5-week-old survivors ( Fig. 3e ), an indication of severe cardiac stress [24] . 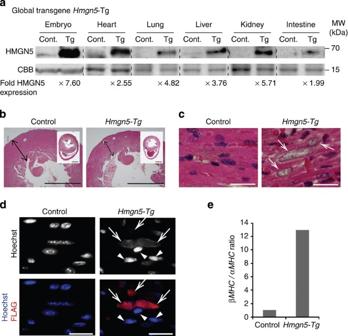Figure 3: Cardiac defects in transgenic mice globally overexpressing HMGN5. (a) Western blots show upregulated HMGN5 expression in all tissues of newbornHmgn5-Tg (Tg) but not in Floxed (Cont.) mice. Coomassie blue (CBB) indicate equal protein loadings. (b) Thinning of cardiac walls and (c,d) Enlarged nuclei showing decompacted chromatin (arrows) in the heart of 3-week-oldHmgn5-Tg mice. FLAG-positive cells indicate expression of FLAG–HMGN5 (arrows). Arrowhead point to FLAG-negative cells. Scale bar,b: 1 mm;c,d: 20 μm. (e) Elevated β/α myosin heavy chain (MHC) transcripts ratio indicate cardiac stress in 5-week-oldHmgn5-Tg mice. Three mice of each genotype were analyzed. Figure 3: Cardiac defects in transgenic mice globally overexpressing HMGN5. ( a ) Western blots show upregulated HMGN5 expression in all tissues of newborn Hmgn5 -Tg (Tg) but not in Floxed (Cont.) mice. Coomassie blue (CBB) indicate equal protein loadings. ( b ) Thinning of cardiac walls and ( c , d ) Enlarged nuclei showing decompacted chromatin (arrows) in the heart of 3-week-old Hmgn5 -Tg mice. FLAG-positive cells indicate expression of FLAG–HMGN5 (arrows). Arrowhead point to FLAG-negative cells. Scale bar, b : 1 mm; c , d : 20 μm. ( e ) Elevated β/α myosin heavy chain (MHC) transcripts ratio indicate cardiac stress in 5-week-old Hmgn5 -Tg mice. Three mice of each genotype were analyzed. Full size image To test whether indeed, the upregulation of HMGN5 can lead to heart dysfunction, we generated mice overexpressing HMGN5 only in the heart ( Hmgn5 -hTG), using mice expressing Cre-recombinase driven by α-MHC promoter, which is induced at E11.5 and remains active after birth. Similar to the global transgenic mice, Hmgn5 -hTG mice, which overexpress HMGN5 only in the heart, showed robust HMGN5 expression ( Fig. 4a ) and seemed normal at birth. Similar to the Hmgn5 -TG mice, these mice did not thrive and 80% of the Hmgn5 -hTG died within 12 weeks of birth ( Fig. 4b ). Magnetic resonance imaging (MRI) of 9-week-old Hmgn5 -hTG mice revealed significant atrial and ventricular enlargement, and thinning of the ventricular walls ( Supplementary Fig. 4d ), which were also seen in excised hearts and in histology sections ( Fig. 4c,d ). Both hematoxylin and eosin and immunofluorescence staining revealed that the heart of the Hmgn5 -hTg mice contained cardiomyocytes with large nuclei showing decondensed chromatin and FLAG, indicating HMGN5 expression ( Fig. 4e ). The heart of adult, but not newborn Hmgn5 -hTG mice showed signs of cardiac stress as indicated by a significant increase in the β-MHC to α-MHC messenger RNA ratio ( Fig. 4f ) and the presence of increased fibrosis in the heart wall [25] ( Supplementary Fig. 4f ). Hmgn5 -hTG mice showed a >50% decrease in the ventricular ejection fraction ( Supplementary Fig. 4e ), a decrease in stroke volume and significant increase in end diastolic and systolic volumes ( Supplementary Table 1 ); all these are indications of a decrease in the ability of the heart to pump blood. The reduced ejection fraction in the hearts promoted the formation of severe atrial thrombi ( Supplementary Fig. 4g ) leading to the mortality of these mice. 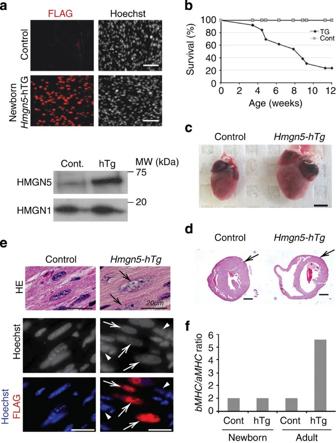Figure 4: Cardiac defects in heart-specific HMGN5 transgenic mice. (a) Elevated expression of HMGN5 protein in the heart of newbornHmgn5-hTg mice. Immunofluorescence (top panel) shows robust expression of the FLAG–HMGN5 in most cells. Bottom panels shows Westerns. HMGN1 serves as loading control. Scale bar, 50 μm (b) Decreased survival ofHmgn5-hTg mice. (c) Enlarged heart in 5-week-oldHmgn5-Tg mice. Scale bar, 2.5 mm. (d) Thinning of cardiac walls in 5-week-oldHmgn5-hTg mice. Scale bar, 1 mm. (e) Enlarged nuclei showing decompacted chromatin (arrows) in the heart of 5-week-oldHmgn5-hTg mice. Arrows point to cells expressing FLAG–HMGN5 and show large nuclei with decompacted chromatin that stain poorly with Hoechst; arrowheads point to cells devoid of FLAG which show smaller nuclei and compact chromatin. Scale bar, 20 μm (f) β/α-myosin heavy chain (MHC) transcripts ratios indicate cardiac stress in 5-week-old adult, but not in newborn transgenicHmgn5-hTg mice. Figure 4: Cardiac defects in heart-specific HMGN5 transgenic mice. ( a ) Elevated expression of HMGN5 protein in the heart of newborn Hmgn5 -hTg mice. Immunofluorescence (top panel) shows robust expression of the FLAG–HMGN5 in most cells. Bottom panels shows Westerns. HMGN1 serves as loading control. Scale bar, 50 μm ( b ) Decreased survival of Hmgn5 -hTg mice. ( c ) Enlarged heart in 5-week-old Hmgn5 -Tg mice. Scale bar, 2.5 mm. ( d ) Thinning of cardiac walls in 5-week-old Hmgn5 -hTg mice. Scale bar, 1 mm. ( e ) Enlarged nuclei showing decompacted chromatin (arrows) in the heart of 5-week-old Hmgn5 -hTg mice. Arrows point to cells expressing FLAG–HMGN5 and show large nuclei with decompacted chromatin that stain poorly with Hoechst; arrowheads point to cells devoid of FLAG which show smaller nuclei and compact chromatin. Scale bar, 20 μm ( f ) β/α-myosin heavy chain (MHC) transcripts ratios indicate cardiac stress in 5-week-old adult, but not in newborn transgenic Hmgn5 -hTg mice. Full size image Lamina disruption in adult but not newborn HMGN5 transgenics Although both Hmgn5 -TG and Hmgn5 -hTG mice seemed normal at birth, newborn cardiomyocytes expressing exogenous HMGN5 showed decompacted chromatin, just like in adult mice ( Fig. 5a–d ). Thus, in newborn mice, the cardiomyocytes that do not overexpress HMGN5 show the DNA and the heterochromatin histone mark H3K9me3 localized to densely staining chromocenters, while the cardiomyocytes that do overexpress HMGN5 show diffuse DNA stain, and the H3K9me3 signal is not prominently localized to chromocenters ( Fig. 5a,c,e ), although the amount of H3K9me3 is not affected ( Supplementary Fig. 4b,c ). 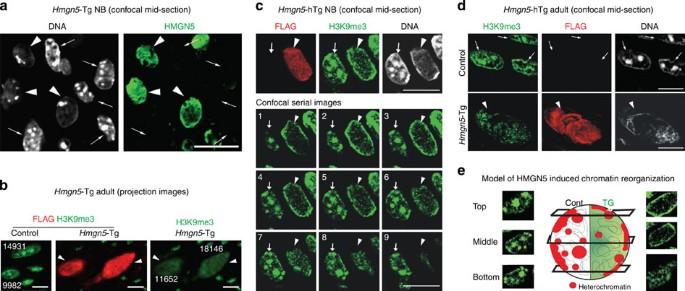Figure 5: Chromatin decompaction in both newborn and adult HMGN5 mice, but nuclear enlargement only in adults. (a–d) In bothHmgn5-Tg andHmgn5-hTg mice, chromatin decompaction is seen in both newborn (NB) and adult cardiomyocytes-overexpressing HMGN5 (arrowheads), but significant nuclear enlargement only in cells from adults. H3K9me3 or DNA (Hoechst), shows significant chromatin decompaction in FLAG–HMGN5-expressing cells. HMGN5 (a) Confocal mid-section images from the new born (NB) transgenic mice, which express HMGN5 globally (Hmgn5-Tg). (b) Confocal mid-section images from the adult transgenic mice, which express HMGN5 globally (Hmgn5-Tg). The numbers adjacent to individual nuclei are arbitrary GFP fluorescence units obtained by quantifying the total fluorescence with Nikon Elements software. (c) Top: confocal mid-section images of heart section from newborn (NB) heart-specific HMGN5 transgenic mice (Hmgn5-hTg). Shown are adjacent cells that either do (arrowhead), or do not (arrow) express FLAG–HMGN5. Bottom: confocal serial images of the cells shown in top. (d) Chromatin decompaction in adultHmgn5-hTg heart. (e) Model of HMGN5-induced chromatin reorganization showing loss of heterochromatin throughout the nucleus. Scale bars, 10 μm. Figure 5: Chromatin decompaction in both newborn and adult HMGN5 mice, but nuclear enlargement only in adults. ( a – d ) In both Hmgn5 -Tg and Hmgn5 -hTg mice, chromatin decompaction is seen in both newborn (NB) and adult cardiomyocytes-overexpressing HMGN5 (arrowheads), but significant nuclear enlargement only in cells from adults. H3K9me3 or DNA (Hoechst), shows significant chromatin decompaction in FLAG–HMGN5-expressing cells. HMGN5 ( a ) Confocal mid-section images from the new born (NB) transgenic mice, which express HMGN5 globally ( Hmgn5 -Tg). ( b ) Confocal mid-section images from the adult transgenic mice, which express HMGN5 globally ( Hmgn5 -Tg). The numbers adjacent to individual nuclei are arbitrary GFP fluorescence units obtained by quantifying the total fluorescence with Nikon Elements software. ( c ) Top: confocal mid-section images of heart section from newborn (NB) heart-specific HMGN5 transgenic mice ( Hmgn5 -hTg). Shown are adjacent cells that either do (arrowhead), or do not (arrow) express FLAG–HMGN5. Bottom: confocal serial images of the cells shown in top. ( d ) Chromatin decompaction in adult Hmgn5-h Tg heart. ( e ) Model of HMGN5-induced chromatin reorganization showing loss of heterochromatin throughout the nucleus. Scale bars, 10 μm. Full size image While chromatin decompaction was obvious in both newborn and adult HMGN5-overexpressing nuclei, nuclear enlargement and lamina changes were observed only in the nuclei of adult mice ( Supplementary Fig. 6 ). In newborns, the fluorescence intensity of lamina in cardiomyocytes showing decondensed chromatin was similar to that of adjacent cells in which the chromatin was condensed ( Fig. 6a ), suggesting that upregulation of HMGN5 levels, which commenced during embryogenesis, did not have noticeable effects on nuclear size or lamina integrity. Likewise, electron microscopy reveals the presence of the lamina underlying the inner nuclear membrane in the nuclei of both control and Hmgn5 -hTg newborn littermates, in spite of the visible differences in the compaction of the chromatin adjacent to the lamina ( Fig. 6c,d , and Supplementary Fig. 5 ). In contrast, in adult Hmgn5 -hTg mice, the lamin A/C immunofluorescence in the large nuclei showing de-compact chromatin was weaker than that seen in smaller nuclei with compact chromatin ( Fig. 6b ). Likewise, electron microscopy revealed an intact lamina in the nuclei of adult control mice, but not in the nuclei of their Hmgn5 -hTg littermates that lacked compacted heterochromatin. In these nuclei, the lamina underlying the inner nuclear membrane was either absent or discontinuous and disrupted ( Fig. 6c,d , and Supplementary Fig. 5 ). Thus, although the chromatin is decompacted in both newborn and adult mice, increased nuclear size and lamina disruption is seen only in the cardiomyocytes of adult mice. 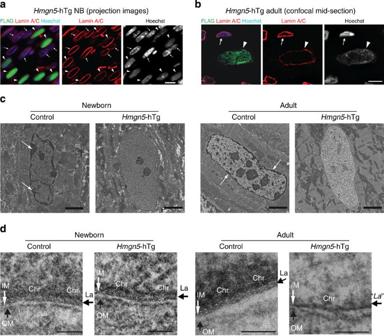Figure 6: Chromatin decompaction in both newborn and adult HMGN5 transgenic cardiomyocytes, but lamina abnormalities seen only in adults. (a) Immunofluorescence reveals intact lamina in cardiomyocytes of newborns regardless whether they do or do not express HMGN5 and their chromatin is, or is not, decompacted. Arrows and arrowheads point to cells with compact and decompact chromatin, respectively.(b) Immunofluorescence reveals weaker staining lamina and in 5-week-old adult cardiomyocytes showing enlarged nuclei and decompacted chromatin. (c) Electron micrograph showing compact heterochromatin (arrows) in control cardiomyocytes and decompacted chromatin in both newborn and adultHmgn5-hTg. (d) Disrupted lamina in adult, but not newbornHmgn5-hTg cardiomyocytes. The lamina (La) is outlined by dashed lines, outer nuclear membrane (OM) and inner nuclear membrane (IM), are indicated by arrows. “La” points to the path of the missing lamina in adultHmgn5-Tg. Scale bars,a,b: 10 μm;c:2 μm;d: 100 nm. Chr: chromatin. Figure 6: Chromatin decompaction in both newborn and adult HMGN5 transgenic cardiomyocytes, but lamina abnormalities seen only in adults. ( a ) Immunofluorescence reveals intact lamina in cardiomyocytes of newborns regardless whether they do or do not express HMGN5 and their chromatin is, or is not, decompacted. Arrows and arrowheads point to cells with compact and decompact chromatin, respectively. ( b ) Immunofluorescence reveals weaker staining lamina and in 5-week-old adult cardiomyocytes showing enlarged nuclei and decompacted chromatin. ( c ) Electron micrograph showing compact heterochromatin (arrows) in control cardiomyocytes and decompacted chromatin in both newborn and adult Hmgn5 -hTg. ( d ) Disrupted lamina in adult, but not newborn Hmgn5 -hTg cardiomyocytes. The lamina (La) is outlined by dashed lines, outer nuclear membrane (OM) and inner nuclear membrane (IM), are indicated by arrows. “La” points to the path of the missing lamina in adult Hmgn5 -Tg. Scale bars, a , b : 10 μm; c :2 μm; d : 100 nm. Chr: chromatin. Full size image Changes in lamina organization can lead to changes in transcription [26] , [27] , [28] . The transcription profile of the hearts taken from newborn Hmgn5 -hTg mice was indistinguishable from that of control siblings ( Fig. 7a , left panel), supporting our observation that Hmgn5 -hTg mice are born with functionally normal hearts and intact nuclear lamina. In the hearts of adult Hmgn5 -hTg mice, the expression of 495 genes was affected, ( Fig. 7a , right); the genes affected were not involved in heart function, suggesting that the transcriptional changes are related to changes in nuclear lamina organization rather than to disruption of heart-specific transcriptional pathways ( Fig. 7a , Supplementary Table 2 ). 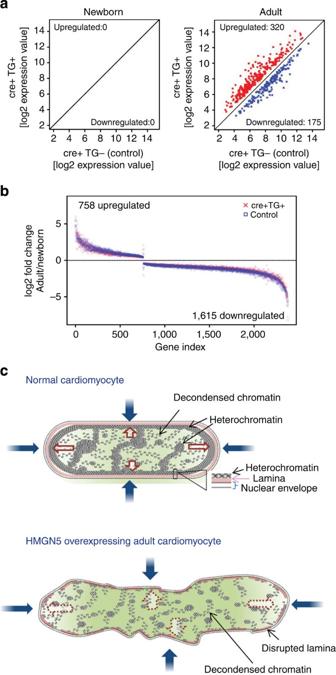Figure 7: Expression analyses. (a) Changes in expression profiles in the heart of newborn and a 5-week-old adultHmgn5-hTg mice (cre+ TG+) with respect to controls (cre+ TG−). While 495 genes were found to be significantly differentially expressed in adult, no gene was identified in newborn mice. (b) HMGN5-mediated chromatin decompaction does not alter the developmentally related changes in cardiac gene expression. Shown are differences between newborn and 3-week-old mice in the expression profile for 2,379 genes in either control orHmgn5-hTg mice. (c) Model depicting a role for heterochromatin in enhancing the mechanical stability of the nucleus. Heterochromatin provides structural support to the nuclear lamina, thereby enhancing its ability to withstand the mechanical stress. In tissue culture cells, chromatin decompaction decreases nuclear sturdiness and elasticity and can lead to blebbing. In cardiomyocytes, heterochromatin provides structural support to the nuclear lamina, thereby enhancing its ability to withstand the mechanical forces of the continuously beating heart. Loss of heterochromatin reduces the ability of the lamina to support the nuclear envelope, decreases nuclear sturdiness and leads to disruption of the nuclear lamina. The transgenic mice develop dilated cardiomyopathy that leads to death. Blue arrows represent external forces acting on the nucleus; red arrows represent opposing forces generated within the nucleus. Figure 7: Expression analyses. ( a ) Changes in expression profiles in the heart of newborn and a 5-week-old adult Hmgn5 -hTg mice (cre+ TG+) with respect to controls (cre+ TG−). While 495 genes were found to be significantly differentially expressed in adult, no gene was identified in newborn mice. ( b ) HMGN5-mediated chromatin decompaction does not alter the developmentally related changes in cardiac gene expression. Shown are differences between newborn and 3-week-old mice in the expression profile for 2,379 genes in either control or Hmgn5 -hTg mice. ( c ) Model depicting a role for heterochromatin in enhancing the mechanical stability of the nucleus. Heterochromatin provides structural support to the nuclear lamina, thereby enhancing its ability to withstand the mechanical stress. In tissue culture cells, chromatin decompaction decreases nuclear sturdiness and elasticity and can lead to blebbing. In cardiomyocytes, heterochromatin provides structural support to the nuclear lamina, thereby enhancing its ability to withstand the mechanical forces of the continuously beating heart. Loss of heterochromatin reduces the ability of the lamina to support the nuclear envelope, decreases nuclear sturdiness and leads to disruption of the nuclear lamina. The transgenic mice develop dilated cardiomyopathy that leads to death. Blue arrows represent external forces acting on the nucleus; red arrows represent opposing forces generated within the nucleus. Full size image The switch from neonatal to adult cardiac function involves major changes in gene expression and can be disrupted by factors that affect epigenetic regulatory mechanisms such as histone modifying enzymes and ATP-dependent chromatin remodelers [29] , [30] . In both wild-type and Hmgn5 -hTg mice the expression of 2,379 genes was changed during heart maturation; of these all but 6 genes were similarly regulated ( Fig. 7b , Supplementary Table 3 ), further evidence that cardiac gene expression in young mice and the cardiac developmental programme is not significantly impacted by the elevated HMGN5 levels. Changes in nuclear lamina are known to alter nuclear structure and chromatin organization [6] , [9] , [26] , [28] , [31] ; we now show that in turn, global changes in heterochromatin affect the properties of the lamina, a finding supported by the previous observation that loss of methyltransferases involved in heterochromatinization leads to lamina disorganization [32] . Studies with yeast cells that lack a distinct lamina suggest that a functional link between the nuclear envelope and chromatin components is a fundamental property of eukaryotic cells [12] , [13] , [33] . The integrity of the lamina and its ability to dampen and withstand the deleterious impact of mechanical forces that can affect chromatin dynamics and gene expression are particularly important to cardiac cells, which are continuously exposed to significant mechanical stress under normal conditions [20] , [34] , [35] , [36] , [37] . Our studies with cells grown in tissue culture and with transgenic mice reveal that chromatin decompaction weakens the mechanical properties of the nucleus, leading to a phenotype similar to that seen in cells and mice with defects in lamina components [6] , [8] , [23] , [38] , [39] . Tissue culture cells with defective lamina show decrease rigidity and elasticity and nuclear blebbing; all these characteristics are also seen in the cells with decompacted chromatin ( Fig. 1 ). Furthermore, our analyses of Lmna −/− cells indicate that HMGN5-mediated chromatin decompaction further weakens the nuclear sturdiness of the Lmna −/− cells, suggesting that heterochromatin and lamina synergistically reinforce the mechanical sturdiness of the nucleus. The phenotype of the HMGN5 transgenic mice resembles the cardiac phenotype of Lmna −/− mice, which lack lamin A/C (ref. 23 ). Both Hmgn5 transgenes and Lmna −/− mice seem normal at birth but their growth rate is retarded, and the nuclei of their cardiomyocytes are enlarged, misshaped and show altered heterochromatin organization. The heart of both adult Lmna −/− and HMGN5 transgenic mice has thinner ventricular walls; their cardiac function is impaired leading to death by 8–10 weeks of age. Mutations in lamina components can induce global chromatin reorganization and gene relocation without necessarily causing major changes in transcription [40] . The major pathophysiological mechanism of the Lmna −/− mice is inability of the cardiomyocyte nucleus to withstand the extracellular forces transmitted through the cytoskeleton [23] . We find that in HMGN5 transgenic mice, in which the chromatin was decompacted during embryogenesis, the size of the nucleus and the lamina underlining the inner nuclear membrane seems normal in newborn ( Fig. 6 , Supplementary Fig. 6 ). However, in adult cardiomyocytes of these mice, the nuclear size is drastically increased and the lamina is disrupted ( Fig. 5 , Supplementary Figs 5 and 6 ). Taken together with the experiments done with tissue culture cells, the results suggest that the cardiac phenotype observed in the HMGN5 mice is a consequence of defects in the transduction of mechanical forces to the nucleus. We suggest that the targeting of heterochromatin to the nuclear periphery, an evolutionarily conserved process [41] , serves not only to position repressed genes, but also to enhance the ability of the nuclear lamina to reinforce the structural integrity of the nucleus ( Fig. 7c ). Our findings reveal a structural role for chromatin that is not directly related to its known genetic functions, and reemphasize the functional relevance of the spatial organization of chromatin in the nucleus. Tissue culture cells MEF was established in our laboratory [42] . NIH/3T3 and HeLa cells were purchased from ATCC. They were grown in Dulbecco modified Eagle medium (DMEM) containing 10% foetal bovine serum under standard conditions. CAT413 cells, a mouse thyroid adenoma cell line, were a kind gift from Dr Shioko Kimura (NCI, NIH). This cell line was grown in DMEM/F-12 containing 10% foetal bovine serum. MEFs prepared from Lmna −/− and their littermate Lmna +/+ mice [19] were a gift from Drs T. Misteli and N. Kubben, (NCI, NIH). Shrinking and swelling experiments Nuclei were isolated as described [20] , with minor modifications. Briefly, NIH 3T3 cells were plated at 1 × 10 6 per 100-mm diameter dish the day before transfection. The cells were transfected by Lipofectamin 2000 (Invitrogen) with 24 μg of either GFP–HMGN5 or GFP–HMGN5-SE. The cultures were fed with fresh medium after 5 h of transfection. After 48 h of transfection, cells were washed with phosphate buffered saline (PBS) twice and with 10 mM HEPES (pH 7.5) containing 1 mM dithiothreitol (DTT) (Sigma-Aldrich, St Louis, MO, USA). Cells were scraped with 200 μl of the HEPES/DTT solution and transferred into centrifuge tube. After 10 min incubation on ice, cell suspensions were sheared in a Dounce homogenizer by a single stroke. A 0.2 volume of 5 × STKMC (1.25 M sucrose, 250 mM Tris, pH 7.5, 125 mM KCl, 15 mM MgCl2, 15 mM CaCl2, 10 μg ml −1 each of pepstatin and leupeptin; Sigma-Aldrich) was added to the cell lysate and incubated for 10 min on ice. A 1.93 volume of 2.3 M sucrose in TKMC (50 mM Tris, pH 7.5, 25 mM KCl, 3 mM MgCl2, 3 mM CaCl2, 2 μg ml −1 each leupeptin and pepstatin) was added to the cell lysate suspension to adjust the sucrose concentration to 1.6 M. A total of the 1.6 M STKMC cell suspension was layered onto a 150 μl cushion of 2.3 M STKMC and spun at 166,000 g in an Optima ultracentrifuge (Beckman Coulter). Nuclei were re-suspended in 100 μl TKMC for condenced state or 100 μl of 10 mM Tris (pH7.5) for swelling. To shrink the swollen nuclei, 0.2 volumes of 5 × TKMC were added and incubated for 20 min. Nuclear images were taken by Zeiss LSM780 confocal microscopy (Carl Zeiss Inc, Thornwood, NY, USA) and the sizes of nuclei were measured by ZEN imaging software. Exposure of cells to fluid mechanical shear NIH 3T3 cells were plated at 1 × 10 6 per 100-mm diameter dish the day before transfection. The cells were transfected by Lipofectamin 2000 with total 24 μg of DNA containing either 12 μg each of GFP–HMGN5 (ref. 14 ), CFP–NLS, or 12 μg each of GFP–HMGN5-SE [14] and mCherry–NLS, as recommended by the manufacturer. Expression vector for mCherry–NLS was constructed by inserting NLS encoding oligonucleotide between NheI and AgeI site of pmCherry–C2 (Clontech). CFP–NLS was constructed by adding NLS between NheI and XhoI site of pECFP-N1 (Clontech). After 5 h of transfection, the cultures were fed with fresh medium. After 48 h of transfection, cells were harvested by trypsin treatment and dissolved in PBS. Aliquots containing 1 × 10 6 of each transfected cell type were mixed in a 15 ml Falcon tube, sedimented at 300 g and re-suspended in 1 ml of 0.1 × PBS and transferred into 1.5 ml centrifuge tube. Using 1 ml syringe, the cell were repeatedly passed through a 26 G needle, at a rate of five passages in 1 min. After each 10 passages, 50 μl of cell suspension was collected, fixed by 3.7% formalin and the number of red and blue nuclei remaining was determined with a Nikon Eclipse E800 microscope using the NIS-Elements AR3.10 software. Atomic force microscopy The instrument used was a commercial AFM (Bioscope-Catalyst with Nanoscope-5 controller, Bruker-Nano, Santa Barbara, CA, USA) on top of an Olympus IX-71 inverted microscope. The AFM is equipped with fluorescence optics for co-localized optical and AFM imaging and manipulation. Young’s moduli and viscoelastic parameters were determined by nanoindentation. The indentation cantilevers had nominal stiffness of 0.01 N m −1 (MSCT-C, Bruker-Nano) and had a 5 μm polystyrene sphere in place of the probe to minimize cell damage that may be caused by sharp probes. The actual stiffness of each cantilever used was measured using the thermal tuning method as provided by the instrument software. Mixed population of cells (control and HMGN5 overexpressing cells) was plated on glass-bottom Petri-dishes coated with gelatin. The plating densities were kept at 1 × 10 4 cells per 50 mm dish, so as to avoid cell confluence. The AFM probe was centred above the cell nucleus using a 50 × objective. Nanoindentations were then performed at an array of points on a grid that covered the whole cell, including points on the glass substrate. The indentation procedure acquired ‘force–volume’ data, namely force–distance curves along with an approximate height map of the cell topography. The latter makes available the sample thickness needed to correct for the effect of the rigid substrate on the apparent elasticity. A total of five sets of data were collected on different sample preparations on different dates. One probe was used on each set. A total of about 50 undamaged cells from each category were analyzed. Indentations were performed at ~10 μm s −1 . To avoid damage, the cells were indented by not more than half of their thickness. To examine whether HMGN5 overexpression alters the viscoelastic response of the cells, we measured the effect of indentation rate on the cell elasticity. Cells were indented at three rates with ratios of 1:5:10 with the lowest rate being again ~10 μm s −1 . Data from cells that showed a decrease in elastic modulus with increased indentation rate were rejected as damaged. Data analysis. The forceσdistance curves were exported using the instrument software and analyzed using custom written Matlab (Mathworks) and Mathematica (Wolfram Research) code. Statistical analysis was performed using Origin (OriginLab) and Excel (Microsoft). The force–distance curves were analyzed by fitting the Hertz model [43] for spherical indenter along with the correction for the finite cell thickness over the rigid glass substrate [44] . The fitting procedure gives an estimate of the Young’s modulus from each curve. Among all the curves, we cropped a subset that includes the highest point of the cell, that is, the point above the nucleus. For the data analysis, the data of each curve were truncated so as to limit indentation to half the cell thickness. The data for the different indentation rates were fitted by a power law function across the different rates and the mean slope of the ensemble for control and for HMGN5 cells were compared. Generation and analysis of transgenic animals All mice used were C57BL6 males of the age indicated in the manuscript. Mice were bred in a specific pathogen-free facility with food and water ad libitum . All animal experiments were performed with the approval of Animal Care and Use Committee (ACUC) of the National Institutes of Health (NIH). The full length mouse Hmgn5 complementary DNA (cDNA), containing the entire 5′-untranslated region (UTR) and FLAG tag at the 3′-end was amplified by PCR and inserted between BglII and XhoI sites of the pCALL vector [45] . This vector contains a floxed LacZ cDNA driven by the CAG (a hybrid cytomegalovirus enhancer and chicken beta-actin) promoter, which is highly active in early mouse embryos [45] . The vector was linearized by NotI digestion and injected into fertilized oocytes of C57BL/6 mice. Transgenic mice were produced as described in ref. 46 . Approximately 200 to 500 copies of the CAG-Hmgn5 chimeric gene were injected into fertilized ova at the single-cell stage. Mice were screened for the acquisition of the novel CAG and Hmgn5 sequences by Southern blotting analysis of DNA obtained from tail biopsies [47] using linearized vector. Expression of beta galactosidase in transgenic mice was assessed by LacZ staining of mouse embryos or tails of the adult animals. Embryos were dissected at 10–12.5 day postcoitum and fixed in fixation buffer (2% formaldehyde, 0.2% glutaraldehyde on PBS × 1) for 1 h at 4 °C. Samples were rinsed twice for 5 min in rinsing solution ( 2 mM MgCl 2 , 0.01% sodium deoxycholate, 0.02% NP-40 on 50 mM phosphate buffer pH 7.2) Staining was performed at 37 °C overnight with shaking in X-gal staining solution (2 mg ml −1 X-gal, 2 mM MgCl 2 , 0.01% sodium deoxycholate, 0.02% NP-40, 5 mM K 3 Fe(CN) 6 , 5 mM K 4 Fe(CN) 6 on 50 mM phosphate buffer pH 7.2). For propagating transgenic lines, only mice with strong beta galactosidase staining of the tail were used. Total embryonic excision of LacZ sequence was done by breeding floxed HMGN5-TG mice with SoxCre mice [48] . Two separate mouse lines were produced, propagated and analyzed. Heart-specific excision was performed by breeding floxed HMGN5-TG mice with alpha MHC-Cre mice [49] . One line was propagated. For genotyping, DNA from the tails of embryos or adult mice was extracted by REDExtract-N-Amp tissue PCR kit (Sigma) and amplified using a mix of three primers: forward 5′- TGGCAAAGAATTCCTCGATCG -3′; reverse 1 5′- TGGCTTGGTTTCAGGAATTGG -3′ and reverse 2 5′- GGTTTTCCCAGTCACGACGTT -3′ at an annealing temperature of 56 °C. REDExtract-N-Amp PCR Ready Mix (Sigma) was used for the PCR reactions. MRI imaging 9- to 11-week-old mice were used for MRI. MRI experiments were performed in a 7.0 T, 16-cm horizontal Bruker MR imaging system (Bruker, Billerica, MA, USA) with Bruker ParaVision 4.0 software. Mice were anesthetized with 1.5–3% isoflurane and imaged with electrocardiogram, temperature and respiratory detection using a 38 mm Bruker birdcage volume coil. Magnevist (Bayer HealthCare, Montville, NJ, USA) diluted 1:10 with sterile 0.9% saline was administered intravenously at 0.3 mmol Gd kg −1 . T1-weighted gradient echo cine images of the heart were acquired in short axis from base to apex (six slices) with the following parameters: repetition time TR=10 to 11 ms, echo time TE=3.4 ms, 10 to 13 frames, 30 degree flip angle, 3–4 averages, 1.0 mm slice thickness, 2.8 to 3.0 cm field of view, 256 × 256 matrix, respiratory and ECG gated. Cardiac MRI data was processed to determine ejection fractions, ventricular volumes and associated functional parameters using CAAS-MRV-FARM software (Pie Medical Imaging, the Netherlands.) Imaging experiments were conducted following institutional animal care and use guidelines. Histology and immunofluorescence staining Affinity pure antibodies to mouse HMGN1 (ref. 42 ) (1:200 for immunofluorescence; 1:1,000 for Westerns) and mouse HMGN5 (ref. 50 ; 1:200 for immunofluorescence; 1:1,000 for Westerns) were prepared in our laboratory. Commercial antibodies Anti-Histone H3 K9me3 (EMD Millipore, #07-442), Anti-Histone H3 K9me2 (Cell Signaling Technology, #9753), Anti-Histone H3 K27me3 (Active Motif, 39155), Anti-LaminA/C (Cell signaling Technology, #4777S), Anti-LaminA/C (Epitomics, #2921-1), Anti-LaminB (Santa-Cruz, #sc-6217), Anti-FLAG (Sigma-Aldorich, #F1804) were used at 1:200 for immunofluorescence and 1:1,000 for Westerns. Mouse tissues and embryos were fixed in 10% formalin solution (Sigma-Aldrich), paraffin sections were examined either by staining with HE by Masson’s Trichrome or by immunofluorescent staining [51] . Microscopy Projection images were collected using a Nikon NIS-Elements AR 3.10 system mounted on a Nikon Eclipse E800 microscope (Nikon). Confocal images were collected using a Zeiss LSM 510 system mounted on a Zeiss Axiovert 200 M microscope (Carl Zeiss Inc, Thornwood, NY, USA) using an oil immersion Plan-Apochromat × 63/1.4 differential interference contrast objective lens. Z-stacked images acquired on the DeltaVision Personal system (Applied Precision Inc, Issaquah, WA, USA) were post processed using Image-Pro Plus software (MediaCybernetics Inc, Bethesda, MD, USA) version 6.3. Electron microscopy The tissue sample preparation for the electron microscopy analysis was described previously [52] . Briefly, mouse heart tissues were fixed in 0.1 M sodium cacodylate buffer, pH7.4, containing 4% formaldehyde and 2% glutaraldehyde. Post fixation was done in 1% osmium tetroxide in same buffer. The tissues were stained in 0.5% uranyl acetate in 0.1 M acetate buffer, pH 4.5 and dehydrated in a series of graded ethanol (for example, 35, 50, 70, 95 and 100%) and 100% propylene oxide, infiltrated in an equal mixture of propylene oxide and epoxy resin overnight and embedded in epoxy resin. The epoxy resin was cured in 55 °C oven, and 80- to 90-nm thin sections were cut and mounted on copper grids, which were stained in uranyl acetate and lead citrate. The grids were examined with a Hitachi H7600 electron microscope operated at 80 kV and digital images were taken with a CCD camera (AMT, Danvers, MA, USA). Western blot analysis Whole-cell lysates were prepared in 1 × SDS–PAGE sample buffer (Bio-Rad) supplemented with protease inhibitors and boiled for 15 min. Tissue lysates were prepared by homogenization in ice cold RIPA buffer (20 mM HEPES, pH 7.0, 300 mM NaCl, 10 mM KCl, 1 mM MgCl2, 20% glycerol, 0.5% Triton X-100, 0.5 mM DTT, complete protease inhibitor cocktail and 1 mM orthovanadate), incubated at 4 °C for 30 min and sedimented at 13 K for 15 min. The supernatants were fractionated on 10% pre-cast criterion gels, transferred by semi-dry method to polyvinylidene difluoride membrane, blocked with non-fat milk in PBS, probed with antibodies and detected by chemiluminiscent using ECL Plus according to manufacturer’s (Amersham) recommendations. Antibodies and their dilutions are described above. Uncropped versions of blots are presented in Supplementary Fig. 7 . RNA isolation, RT–PCR and expression array analysis Samples for genotyping were collected from the left ventricle and RNA was prepared with TRIzol reagent according to manufacturer’s protocol following further purification with RNeasy kit (Qiagen). For RT–PCR analysis 500 ng of RNA were used for cDNA synthesis by iScript kit (Bio-rad). Equal amount of cDNA was loaded for RT–PCR reactions with Power SYBR Green power mix (Applied Biosystems). Reactions and measurements were performed using AB 7900HT Fast Real Time PCR system and software. Primer sequences for Myh6 (α-MHC) and Myh7 (β-MHC) were previously published [53] . For expression arrays analysis, RNA was cleaned up by RNeasy kit with on-column DNaseI treatment. Expression array analysis was performed on Affymetrix Mouse GeneChips 430 2 (430v2). Hybridization of biotin-labelled cRNA fragment to Mouse Genome 430 2.0 array, washing, staining with streptavidin–phycoerythrin (Molecular Probes) and signal amplification were performed according to the manufacturer’s instructions at the Laboratory of Molecular Technology (LMT, Frederic, NCI). Mouse 430_2.0 Genome Genechip arrays contain 45,101 probe sets, which were associated with ~20,000 genes using information provided by the Jackson Laboratory ( http://www.informatics.jax.org/ ). All data is MIAME compliant and has been deposited in a MIAME compliant database (GEO_ID). Hybridization intensity raw data (*.CEL files) were processed using the R computing environment ( http://www.r-project.org/ ) version 2.10.1, (R Development Core Team 2009) Bioconductor packages ( http://www.bioconductor.org/ ) [54] and a collection of custom Perl scripts. Normalized gene expression values were generated by the Robust Multi-Array Averaging method using the Bioconductor packages affy [55] and simpleaffy [56] . All analyses were done at the so-called sequence level, that is, data from probes representing the same gene were combined. Statistical differences in gene expression between all samples were determined using the nonlinear Bayes methodology in the Bioconductor package limma [57] . P values were adjusted for multiple testing using Benjamini and Hochberg’s method to control the false discovery rate [58] . Genes with adjusted P values <0.01 were considered to be differentially expressed. All possible pair-wise comparisons between the four samples considered yielded 5,115 differentially expressed genes. Functional analysis was based on overrepresentation of Gene Ontology categories [59] , [60] . Statistical enrichment was quantified using Fisher’s exact test. We report categories with P values adjusted for multiple testing using Benjamini and Hochberg’s method [58] that are <0.05. The array data is available in the GEO database under accession number: GSE63530. How to cite this article: Furusawa, T. et al . Chromatin decompaction by the nucleosomal binding protein HMGN5 impairs nuclear sturdiness. Nat. Commun. 6:6138 doi: 10.1038/ncomms7138 (2015).